Quantal and graded stimulation of B lymphocytes as alternative strategies for regulating adaptive immune responses Lymphocytes undergo a typical response pattern following stimulation in vivo : they proliferate, differentiate to effector cells, cease dividing and predominantly die, leaving a small proportion of long-lived memory and effector cells. This pattern results from cell-intrinsic processes following activation and the influence of external regulation. Here we apply quantitative methods to study B-cell responses in vitro . Our results reveal that B cells stimulated through two Toll-like receptors (TLRs) require minimal external direction to undergo the basic pattern typical of immunity. Altering the stimulus strength regulates the outcome in a quantal manner by varying the number of cells that participate in the response. In contrast, the T-cell-dependent CD40 activation signal induces a response where division times and differentiation rates vary in relation to stimulus strength. These studies offer insight into how the adaptive antibody response may have evolved from simple autonomous response patterns to the highly regulable state that is now observed in mammals. B cells possess multiple activation pathways that help them respond to pathogens. In general, B-cell receptor (BCR) ligation by antigen is not sufficient to drive the B cell to proliferate and differentiate, additional signals are necessary for full activation. These co-stimulatory signals fall into two categories: those associated with innate pathogen recognition and those derived from T cells. Innate signals are typically provided through the Toll-like receptor (TLR) family. Ten members of the TLR family are expressed in mice [1] , [2] , [3] , [4] ; however, their expression patterns are highly cell-type dependent [5] , [6] , [7] . Within the B-cell lineage TLR3, TLR4, TLR7 and TLR9 are found, although TLR3 expression is restricted to marginal zone B cells [6] , [7] . T-cell-dependent signalling requires the interaction of an antigen-specific B cell with an activated T cell that recognizes peptides internalized and presented by the B cell. The T cell provides co-stimulatory signals, including CD40L expression [8] , [9] and secreted cytokines. Perhaps surprisingly, for either mode of stimulation, signals delivered by BCR engagement are not obligatory for B cells to respond, although they do modulate the outcome [10] , [11] , with the BCR serving to attract and focus the co-stimulatory signals to antigen-specific B-cells [12] . As a result, provision of appropriate concentrations of TLR ligands or CD40 (in conjunction with cytokines) can induce proliferation and differentiation of B cells in vitro in the absence of BCR stimulation [10] , [13] , [14] , [15] , [16] . When stimulated in vivo in either a T-dependent (TD) or T-independent (TI) manner, B cells follow the typical pattern of adaptive immunity: most selected cells proliferate, differentiate, stop dividing and die, with a small cohort of long-lived effector and memory cells remaining. Although all B cells are initially similar in their characteristics, heterogeneity emerges after activation, with some B cells becoming plasmablasts, some undergoing isotype switching and others doing both [17] . During TD stimulation, a proportion of cells initiate a germinal centre and eventually give rise to long-lived memory or plasma cells [17] . Given the complexity of cellular environments in lymphoid tissues and germinal centres, cell fate heterogeneity is usually attributed to the variable history and features of each cell. For example, the tissue niche, exposure to a range of soluble and cell-bound signalling ligands, or the affinity of the receptor for the pathogen, all lead to differences in fate determination for each cell [18] , [19] , [20] , effectively by alterations to external signals. In contrast to the view that cell fate is externally directed, recent evidence suggests that internal regulation alone might be sufficient to pattern a typical lymphocyte response. Individual B cells stimulated with CpG DNA and tracked by video microscopy [13] divide 2–5 times before stopping and eventually dying. The generation at which these cells cease to divide—their ‘division destiny’—is inherited from each founder cell and correlated with the size that cell reached before its first division. This pattern suggests that division destiny is a function of the stimulation experienced by the first cell and that epigenetic mechanisms are set in place during this initial period that limit the extent of the ‘division burst’. B cells stimulated by TLR4 ligands or TD stimuli cannot be tracked individually in the same manner as they self-adhere, but when followed as populations by flow cytometry, they exhibit a similar pattern of growth, cessation and death [21] , [22] . Furthermore, individual B cells imaged over a single generation allocate to alternative fates according to a simple pattern of statistical competition [23] . These data suggest that B cells can respond as ‘automatons’ and that only minimal stimulation is required to evoke complex immune response patterning. Here we use quantitative methods [13] , [21] , [23] , [24] to examine the minimal signalling requirements for the canonical pattern of the adaptive immune response in vitro by single stimuli, and extend this analysis to assess differentiation outcomes. We examine three-well-studied B-cell-activating protocols: CD40 ligation as a typical T-cell stimulus, TLR4 stimulation by lipopolysaccharide (LPS) as an external innate signal and TLR9 stimulation, which requires endosomal entry of the ligand CpG. Our results highlight two different mechanisms used by B cells to integrate signals and allocate cells to alternative effector lineages. The two evolutionarily primitive TLR stimuli initiate an all-or-none automatous response, whereas TD stimulation varies times to divide in a graded manner leading to more complex relationships between stimulation strength and differentiation outcomes. TLR9 stimulation invokes a quantal autonomous response B cells stimulated with the TLR9 agonist CpG undergo a limited number of divisions before they stop dividing and eventually die [13] , [22] . This response does not result in isotype switching or the development of dividing antibody-secreting cells (ASCs). B cells dividing in response to CpG follow a simple kinetic pattern, with the time taken to reach the first division averaging around 30 h and times through each subsequent division being more rapid (~10 h). As shown in Fig. 1a , the number of proliferating cells collected from a responding population declines as the CpG concentration is lowered, although a similar pattern of growth, cessation and death is observed. 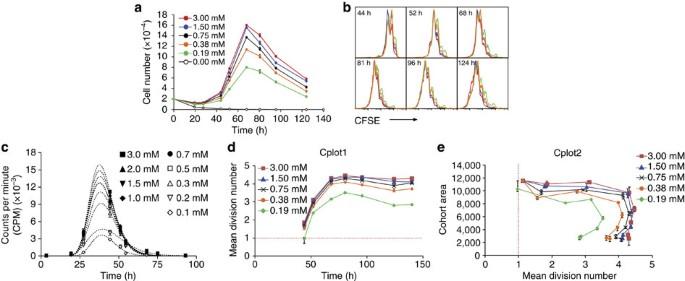Figure 1: Quantitative analysis of CpG stimulation. Naive B cells were labelled with CFSE and stimulated with indicated concentrations of CpG DNA. (a) Measurement of total cell numbers over time in response to CpG titration. Data points=mean±s.e.m. of triplicate cultures. (b) Division progression of B cells was determined by dilution of CFSE. (c) Mean time to first division in response to CpG stimulation was quantified by measuring3H thymidine incorporation during a 1-h pulse in the presence of the cell cycle-inhibitor colcemid. Data points=mean±s.e.m. of triplicate cultures. (d) Cohort analysis was used to measure the mean division number of individual cohorts. Cplot1 were then constructed by plotting data against collection time to visualize the change in maximum division number (division destiny) and division rate with CpG concentration. Red line=intercept with 1 and approximate time to first division. (e) Cohort analysis was used to measure the area of individual cohorts, and therefore number of cells at each time point. Cplot2 was then generated by plotting cohort area against mean division number from Cplot1. Cplot2 was used to approximate changes in death with concentration of CpG. Error bars indanderepresent 95% confidence intervals. All data are representative of three independent experiments. Figure 1: Quantitative analysis of CpG stimulation. Naive B cells were labelled with CFSE and stimulated with indicated concentrations of CpG DNA. ( a ) Measurement of total cell numbers over time in response to CpG titration. Data points=mean±s.e.m. of triplicate cultures. ( b ) Division progression of B cells was determined by dilution of CFSE. ( c ) Mean time to first division in response to CpG stimulation was quantified by measuring 3 H thymidine incorporation during a 1-h pulse in the presence of the cell cycle-inhibitor colcemid. Data points=mean±s.e.m. of triplicate cultures. ( d ) Cohort analysis was used to measure the mean division number of individual cohorts. Cplot1 were then constructed by plotting data against collection time to visualize the change in maximum division number (division destiny) and division rate with CpG concentration. Red line=intercept with 1 and approximate time to first division. ( e ) Cohort analysis was used to measure the area of individual cohorts, and therefore number of cells at each time point. Cplot2 was then generated by plotting cohort area against mean division number from Cplot1. Cplot2 was used to approximate changes in death with concentration of CpG. Error bars in d and e represent 95% confidence intervals. All data are representative of three independent experiments. Full size image We sought to determine which features of proliferation and survival are affected by stimulation strength in this simple system. Figure 1b shows carboxyfluorescein succinimidyl ester (CFSE) division-tracking profiles from different CpG stimulation doses overlaid for the same responding cell population. The position of the peak of proliferation exhibited by the dividing cells is similar, which suggests that stimulation strength regulates the number of cells that initially enter division, but that subsequent division and death are less affected. To test the effect of CpG stimulation strength on time to first division directly, B cells were cultured with different CpG concentrations in the presence of the cell cycle-inhibitor colcemid to allow cells to undergo one round of DNA replication only. The cultures were pulsed with [ 3 H]thymidine for 1 h at regular time intervals [21] , [25] , [26] and the incorporation measured ( Fig. 1c and Supplementary Table S1 ). These data exhibit a lognormal pattern of time of entry to division, as noted for responses to other B- and T-cell stimuli [21] , [25] , [26] . Notably, the mean and s.d. of times to divide are unaffected by the strength of stimulation ( Supplementary Table S1 ). In contrast, the area under these curves is smaller with each reduction in CpG concentration ( Supplementary Table S1 ). This indicates that, as stimulation strength is lowered, the time to first division remains constant, but the proportion of cells that enter division is reduced. To further analyse the quantitative features of division progression, we applied the ‘precursor cohort analysis’ method described previously [24] , [26] , [27] . This method removes the effect of cell expansion from division-tracking data and uses graphical methods to reveal information about the population dynamics of the activated cells. Two graphs are used here: a plot of the average division number of the cohort against collection time (Cplot1) and a plot of the cohort size against mean division number (Cplot2). Cplot1 allows the time to first division and time between subsequent divisions to be estimated [24] , [26] , [27] . Cplot2 provides an indication of the number of cells participating in the response as well as the proportion of cells that die while progressing through divisions. Figure 1d shows Cplot1 for varying levels of CpG stimulation. The mean division number begins to plateau between 60 and 70 h at all concentrations ( Fig. 1d ), consistent with the observed time at which proliferation ceases in these cultures ( Fig. 1a ). Also notable is that the maximum mean division number is lower at lower concentrations, suggesting that CpG stimulus strength regulates the number of divisions that cells ultimately reach. Figure 1e shows Cplot2 for the same data. Here cohort sizes are unchanged after first division, indicating that little cell death occurs until cells reach their destiny division, resulting in a loss of cells at a similar division number. In CPlot2, the reduction in mean division number when death occurs at later time points indicates a survival advantage for cells that have undergone fewer division, a feature also unaffected by concentration of CpG. These data suggest that CpG regulates the strength of the B-cell response in only two ways: first, that increased stimulation increases the proportion of cells in the population that are stimulated above the threshold needed to transit to first division and, second, that the continued progression of these cells to the division destiny limit decreases with lower stimulation strengths, leading to fewer cell divisions overall. Quantal responses to LPS integrate division-linked changes The response of B cells to LPS is also a TLR-dependent mechanism, but is more complex than the response to CpG because many of the dividing cells rapidly differentiate to ASC [11] , [28] , [29] ( Supplementary Fig. S1 ). Quantitative analysis of LPS stimulation shows a similar pattern of growth and division as seen with CpG ( Fig. 2a–f ). As expected, reducing the dose of LPS causes a reduction in cell number after 4 days in culture ( Fig. 2a ) and, in a similar manner to the response to CpG, lowering the stimulation dose increases the proportion of cells remaining undivided, whereas those cells that do divide progress to a similar extent ( Fig. 2b ). 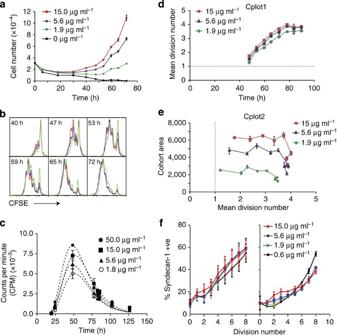Figure 2: Quantitative analysis of LPS stimulation. Naive B cells were labelled with CFSE and stimulated with indicated concentrations of LPS. (a) Measurement of total cell numbers over time in response to LPS titration. Data points=mean±s.e.m. of triplicate cultures. (b) Division progression of B cells was determined by dilution of CFSE. (c) Colcemid plot of mean time to first division in response to LPS stimulation. Data points=mean±s.e.m. of triplicate cultures (d) Cplot1 of cohort analysis of LPS data to visualize the change in maximum division number (division destiny) and division rate with LPS concentration. Red line=intercept with 1 and approximate time to first division. (e) Cplot2 was used to approximate changes in death with concentration of LPS. Error bars indanderepresent 95% confidence intervals (f) Proportion of syndecan-1+cells per division was measured at day 4 in cultures containing CFSE-labelled B cells stimulated with either LPS (left panel) or LPS and IL-4 (right panel). Data points infrepresent the mean and s.e.m. of four replicate samples. All data are representative of four independent experiments. Figure 2: Quantitative analysis of LPS stimulation. Naive B cells were labelled with CFSE and stimulated with indicated concentrations of LPS. ( a ) Measurement of total cell numbers over time in response to LPS titration. Data points=mean±s.e.m. of triplicate cultures. ( b ) Division progression of B cells was determined by dilution of CFSE. ( c ) Colcemid plot of mean time to first division in response to LPS stimulation. Data points=mean±s.e.m. of triplicate cultures ( d ) Cplot1 of cohort analysis of LPS data to visualize the change in maximum division number (division destiny) and division rate with LPS concentration. Red line=intercept with 1 and approximate time to first division. ( e ) Cplot2 was used to approximate changes in death with concentration of LPS. Error bars in d and e represent 95% confidence intervals ( f ) Proportion of syndecan-1 + cells per division was measured at day 4 in cultures containing CFSE-labelled B cells stimulated with either LPS (left panel) or LPS and IL-4 (right panel). Data points in f represent the mean and s.e.m. of four replicate samples. All data are representative of four independent experiments. Full size image Direct measurements confirmed that the mean and variation in time to first division were not affected by the LPS concentration ( Supplementary Table S2 ). However, as seen for CpG stimulation, the total number of cells entering first division became smaller with decreasing LPS concentration ( Fig. 2c and Supplementary Table S2 ). Cplot1 of B-cell responses to LPS produced straight lines consistent with constant division time through successive divisions ( Fig. 2d ). The gradients of regression lines fitted to the data were similar for all concentrations, suggesting that division time is not affected by LPS signal strength ( Fig. 2d ). Figure 2e shows Cplot2 for the same data. Again, as for CpG, the plots are initially parallel with the x axis, indicating little death once division has begun. This pattern ends as cells reach a final division and the cohort area falls progressively due to cell death ( Fig. 2e ). The reduction in the cohort area at first division in lower LPS concentrations is additional evidence that the proportion of cells entering first division is dependent on LPS concentration, as seen for CpG. The differentiation of B cells to ASC in response to LPS provides another variable by which stimulus strength might alter B-cell responses. We measured the appearance of ASC (using syndecan-1 as a marker [29] ), with division for different concentrations of LPS. Figure 2f illustrates that the proportion of syndecan-1 + cells in each division is not significantly affected by concentration. Addition of IL-4 increases the correlation of syndecan-1 with ASC differentiation to over 90% (ref. 29 ). Therefore, we conducted the assays again in the presence of IL-4, yielding identical results ( Fig. 2f ). Thus, by dissecting the contribution of each individual component of an antibody response, we reveal a simple mechanism for the regulation of antibody production in response to LPS: the concentration of LPS affects the proportion of cells that enter the first division and, to a lesser extent, the proportion that progress through subsequent divisions; times to division and rates of ASC differentiation per division remain unchanged. CD40 ligation affects multiple aspects of B-cell responses TD B-cell activation can be mimicked in vitro by stimulating B cells through the CD40 receptor with recombinant CD40L expressed on a cell surface, membrane extracts [30] , [31] , CD40L multimers [32] or agonistic antibodies [33] , [34] . To minimize local stimulation variation for individual cells in the population, we used the soluble αCD40 antibody 1C10 (refs 21 , 22 , 23 , 35 ). In the presence of cytokines such as IL-4 and IL-5, this antibody evokes the typical division-linked isotype switching and differentiation seen following membrane-bound CD40L ligation [36] . To determine the effect of the strength of CD40 stimulation on B-cell responses, a time-series tracking cell proliferation was performed. A dose-dependent increase in proliferation was observed beyond 50 h ( Fig. 3a ). However, in marked contrast to CpG and LPS-stimulated B cells, varying the concentration of αCD40 antibody altered the number of divisions the responding cells progressed through ( Fig. 3b ). 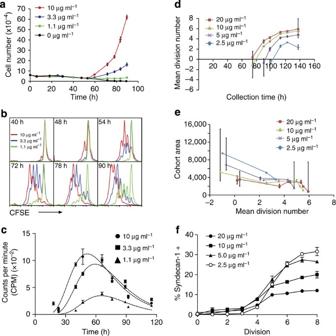Figure 3: Quantitative analysis of CD40 stimulation. Naive B cells were labelled with CFSE and stimulated with indicated concentrations of αCD40 antibody in the presence of constant IL-4. (a) Measurement of total cell numbers over time in response to αCD40 titration. Data points=mean±s.e.m. of triplicate cultures. (b) Division progression of B cells was determined by dilution of CFSE. (c) Colcemid plot of mean time to first division in response to CD40 stimulation. Data points=mean±s.e.m. of triplicate cultures. (d) Cplot1 of cohort analysis of αCD40 data to visualize the change in maximum division number (division destiny) and division rate with αCD40 concentration. Red line=intercept with 1 and approximate time to first division. (e) Cplot2 was used to approximate changes in death with concentration of αCD40. Error bars indanderepresent 95% confidence intervals. (f) Proportion of syndecan-1+cells per division was measured at day 5 in cultures containing CFSE-labelled B cells stimulated with αCD40. Data points represent the mean and s.e.m. of three replicate samples and are representative of three independent experiments. Time-course data (a–e) are representative of four independent experiments. Figure 3: Quantitative analysis of CD40 stimulation. Naive B cells were labelled with CFSE and stimulated with indicated concentrations of αCD40 antibody in the presence of constant IL-4. ( a ) Measurement of total cell numbers over time in response to αCD40 titration. Data points=mean±s.e.m. of triplicate cultures. ( b ) Division progression of B cells was determined by dilution of CFSE. ( c ) Colcemid plot of mean time to first division in response to CD40 stimulation. Data points=mean±s.e.m. of triplicate cultures. ( d ) Cplot1 of cohort analysis of αCD40 data to visualize the change in maximum division number (division destiny) and division rate with αCD40 concentration. Red line=intercept with 1 and approximate time to first division. ( e ) Cplot2 was used to approximate changes in death with concentration of αCD40. Error bars in d and e represent 95% confidence intervals. ( f ) Proportion of syndecan-1 + cells per division was measured at day 5 in cultures containing CFSE-labelled B cells stimulated with αCD40. Data points represent the mean and s.e.m. of three replicate samples and are representative of three independent experiments. Time-course data ( a – e ) are representative of four independent experiments. Full size image This reduction in cell progression could result from a delay in time to first division, an increase in subsequent division times or both. To distinguish between these possibilities, the effect of stimulation on time to first division was measured directly. Fitted lognormal curves show that reducing the concentration of stimulus delayed time to first division and increased the variance ( Fig. 3c and Supplementary Table S3 ). The area also decreased, although, in contrast to CpG and LPS, this may be because the increased time to divide leads to the loss of some cells before entry to division, as previously reported [21] . In Cplot1, the intercept with division one confirms that the average time to first division lengthens as stimulation strength weakens ( Fig. 3d ). However, the plots do not conform to a straight line because of the division number plateau being reached, so the division time for subsequent divisions cannot be estimated. Cplot2 for these data indicate relatively little progressive cell loss as division proceeds ( Fig. 3e ). When the concentration of αCD40 is low, the significant delay in progression through division ( Fig. 3b ) and increased s.d. in entry to first division ( Fig. 3c ) reduce the number of cohorts that record a positive mean division number. In this scenario, an advantage of the cohort method is the ability to fit distributions to the data that extrapolate to negative values ( Fig 3d,e ), allowing additional data points to be obtained. We next examined ASC differentiation per generation and noted that in contrast to LPS-stimulated B cells, reducing the amount of CD40 stimulation led to an increase in the proportion of syndecan-1 + cells measured in each division ( Fig. 3f ). These data reveal that the regulation of proliferation and survival follows a different strategy for the TI and TD stimulus (summarized in Fig. 4 ). 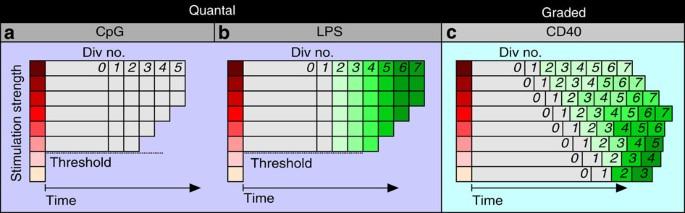Figure 4: Three distinct patterns of proliferation and differentiation for B cells. The two panels on the left (a,b) illustrate the quantal all-or-none stimulation seen with TLR ligation. Different average stimulation doses are illustrated by the vertical heat map (darker being stronger stimulation). Once stimulation is above a threshold, cells proceed to first and subsequent divisions. The times for division are fixed for all levels of stimulation. Stimulation does affect the number of divisions reached and therefore the initiation of cell death. LPS-stimulated cells progressively differentiate to ASC as they divide, illustrated here by the increasing intensity of green. In the right panel (c), the graded response seen for CD40 stimulation is shown. The time to first division is graded by stimulation strength, as is the total number of divisions reached. Here the proportion of cells becoming ASC per division is higher at the lower stimulation strengths, perhaps linking differentiation to time exposed to the stimulus within any single division. Figure 4: Three distinct patterns of proliferation and differentiation for B cells. The two panels on the left ( a , b ) illustrate the quantal all-or-none stimulation seen with TLR ligation. Different average stimulation doses are illustrated by the vertical heat map (darker being stronger stimulation). Once stimulation is above a threshold, cells proceed to first and subsequent divisions. The times for division are fixed for all levels of stimulation. Stimulation does affect the number of divisions reached and therefore the initiation of cell death. LPS-stimulated cells progressively differentiate to ASC as they divide, illustrated here by the increasing intensity of green. In the right panel ( c ), the graded response seen for CD40 stimulation is shown. The time to first division is graded by stimulation strength, as is the total number of divisions reached. Here the proportion of cells becoming ASC per division is higher at the lower stimulation strengths, perhaps linking differentiation to time exposed to the stimulus within any single division. Full size image Quantitative hypothesis testing To further test the conclusions drawn from the above analyses, we used the experimentally designed cyton model of cell proliferation and death [21] , [24] , [25] . This model assumes: (1) competing division and death times in individual cells drawn independently from distinct probability density distributions; (2) redrawing of division and death times in each cell after each division; and (3) a mechanism for the division cessation of a proportion of cells each generation (‘progressor fraction’ or pF). Experimental measurements allow constraints to be introduced into the cyton model that reduce the number of parameters needed. For example, experiments suggest that although first division is a special case, the distributions of division and death times do not change in subsequent divisions. This allows the same pdf to be used for the division and death times of all cells that have proceeded beyond the first division, reducing the number of parameters in the model. In addition, the pF for each generation is known to follow a simple pattern [21] , [22] , so that we use only three free parameters for the pF overall divisions. where is a normal distribution with mean μ and s.d. σ . The parameter γ is a free parameter of the model; thus, in this implementation we have 13 free parameters. When fitting to multiple data sets, such as those obtained at different stimulus concentrations, we have a maximum of 13 free parameters for each concentration. We can, however, constrain some of these parameters to be equal across all concentrations, thus reducing the number of parameters in the fit. We assess the fit quality of models with the Akaike information criterion (AIC), which allows the comparison of multiple models that are not nested; the model that gives the lowest AIC is best. The model was fit to the data for each CpG concentration. ( Fig. 5 and Supplementary Fig. S2 ). We then fit the same data with identical parameter values associated with times to division and death for each concentration but allowing the frequency of cells progressing through divisions to alter, as suggested by experimental evidence ( Fig. 5 and Supplementary Tables S4 and S5 ). This constraint reduced the number of free parameters from 56 to 24 for the entire data set. Although the model with the greatest number of degrees of freedom provided the best fit, the AIC for the constrained model was lower than that for the unconstrained model (2,310 compared with 2,363; Supplementary Table S6 ), supporting the conclusion that division progression is the dominant cell feature affected by CpG stimulation strength. 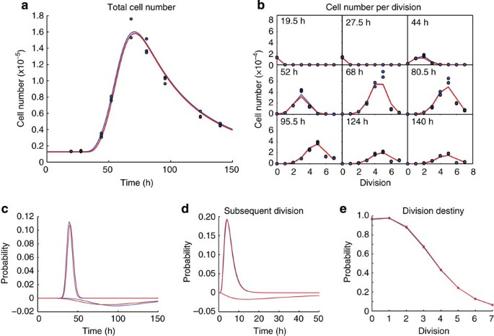Figure 5: Cyton fitting to CpG concentration 3.0 mM. In each case, the blue line show fits obtained from the cyton model with no constraints, whereas the red lines show the fits obtained with all the parameters for death and division times constrained to be equal for all CpG concentrations. (a) Total cell number as a function of time; here the blue points represent triplicate experimental observations. (b) Cell numbers per division at different time points; again the blue points are triplicate experimental observations. (c) Probability density functions for the division times of undivided cells and the negative probability density function of time to die for undivided cells. (d) Probability density functions for the division times of divided cells and the negative probability density function of time to die for divided cells. (e) Probability that the cells are division capable as a function of division. Figure 5: Cyton fitting to CpG concentration 3.0 mM. In each case, the blue line show fits obtained from the cyton model with no constraints, whereas the red lines show the fits obtained with all the parameters for death and division times constrained to be equal for all CpG concentrations. ( a ) Total cell number as a function of time; here the blue points represent triplicate experimental observations. ( b ) Cell numbers per division at different time points; again the blue points are triplicate experimental observations. ( c ) Probability density functions for the division times of undivided cells and the negative probability density function of time to die for undivided cells. ( d ) Probability density functions for the division times of divided cells and the negative probability density function of time to die for divided cells. ( e ) Probability that the cells are division capable as a function of division. Full size image A similar analysis was applied to the LPS data ( Supplementary Fig. S3 and Supplementary Tables S7–S9 ). Here, the AIC suggests that the free fit remains better than that constrained to alter the pF only (1,412 compared with 1,515; Supplementary Table S10 ). However, in these cultures we expect the large proportion of ASC generated to complicate the fitting of a simple model, as the two distinct populations (plasmablasts and lymphoblasts) are likely to have different proliferation and survival features, requiring additional parameters for a complete description. Nevertheless, even assuming identical rates for the two cell types, an excellent fit is possible if only the survival of undivided cells and the parameters associated with the pF are allowed to change ( Supplementary Fig. S3 , Supplementary Tables S7–S9 ). We also note that the unconstrained model fits are achieved by delaying the time to first division in a dose-dependent manner, a result which is not consistent with experimental measurement of this parameter ( Fig. 2c and Supplementary Table S2 ), and thus we can reject the outcome of this fitting. We next used cyton analysis to examine the effects of CD40 stimulation. On the basis of the experimental analysis, we adopted a strategy that allows parameters associated with time to first division to vary with stimulus concentration and compared results with those allowing all parameters to vary ( Fig. 6 , Supplementary Fig. S4 and Supplementary Tables S11–S13 ). Similar to previous analysis, the unconstrained model provides a better fit, but the AIC imply that the constrained model provides the best description of the data (unconstrained AIC-1660; constrained AIC-1639; Supplementary Table S14 ). We compared these fits with one obtained by constraining parameters that provided the best description of the CpG and LPS data (black line Fig. 6 and Supplementary Fig. S4 ), but this analysis was rejected as it returned the highest AIC value of all models (1,700; Supplementary Table S14 ). These analyses support the conclusion that changing pF per division is the dominant effect of altering TLR stimulation strength, whereas changing the times to divide is the dominant outcome of changes to CD40 stimulation strength. 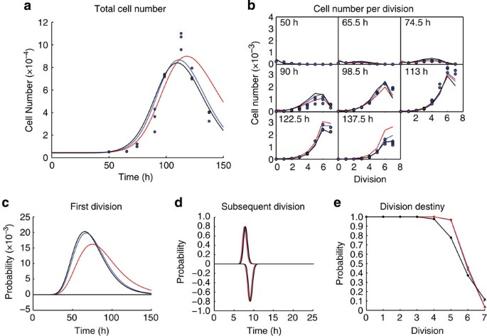Figure 6: Cyton fitting to αCD40 concentration 20 μg ml−1. In each case, the blue lines show fits obtained from the cyton model with no constraints, whereas the black lines show the fits obtained with all the parameters for death and division times constrained to be equal for all αCD40 concentrations, and the red lines show fits obtained where all the parameters associated with times to death and division, apart from time to initial division, are fixed for all concentrations. (a) Total cell number as a function of time; here the points represent experimental observations. (b) Cell numbers per division at different time points; again the points are experimental observations. (c) Probability density functions for the division times of undivided cells and the negative probability density function of time to die for undivided cells. (d) Probability density functions for the division times of divided cells and the negative probability density function of time to die for divided cells. (e) Probability that the cells are division capable as a function of division. Figure 6: Cyton fitting to αCD40 concentration 20 μg ml −1 . In each case, the blue lines show fits obtained from the cyton model with no constraints, whereas the black lines show the fits obtained with all the parameters for death and division times constrained to be equal for all αCD40 concentrations, and the red lines show fits obtained where all the parameters associated with times to death and division, apart from time to initial division, are fixed for all concentrations. ( a ) Total cell number as a function of time; here the points represent experimental observations. ( b ) Cell numbers per division at different time points; again the points are experimental observations. ( c ) Probability density functions for the division times of undivided cells and the negative probability density function of time to die for undivided cells. ( d ) Probability density functions for the division times of divided cells and the negative probability density function of time to die for divided cells. ( e ) Probability that the cells are division capable as a function of division. Full size image B cells possess a complex antigen-binding receptor and an array of additional receptors that modulate their proliferation, survival and differentiation in response to both the concentration and source of stimulation. Together, these regulators offer many potential scenarios for B-cell behaviour in vivo and present a challenge for experimental dissection of the B-cell signal integration program in quantitative terms. Despite the potential complexity, the receptors TLR4 and TLR9, which belong to the innate immune system and are found in many forms of early organisms, including insects, evoke a typical adaptive B-cell response. Perhaps consistent with their primitive origins, we found that these TI responses followed a simple pattern of response. TLR stimulation led B cells into a program that resulted in a regulated, limited division burst, division-linked differentiation (for TLR4) and, when division ceased, the inevitable passage through to programmed cell death. TLR4 stimulation induces more rounds of division, and a much greater rate of differentiation to ASC per division than that seen for TLR9. However, the combined results of our filming studies of proliferation [13] and the quantitative studies here suggest that the autonomous, programmed response emanating from a single stimulated B cell seems fixed. Thus, this cell response can be described as that of an automaton, with entry to the first division emerging as the most important gateway for regulating the generation of lymphoblast and plasmablast cells. The data also reveals that the dose response for these TI ligands is quantal, as the outcome, entry to the response, is all-or-none for individual cells at the first division. These studies raise the question of whether all of the impetus and information for the proliferative response is autonomous and programmed into the first cell. Earlier, we reported the results of experiments where stimulus was removed before cells entering first division, and this led to a reduction in the division destiny and smaller clone sizes [22] . Thus, we conclude that some level of additional stimulation can be acquired within each generation to extend the range of division before cessation. This conclusion may explain why lower concentrations of LPS and of CpG lead to fewer rounds of division, as seen in Figs 1d and 2e . Thus, we argue that the primary features of the adaptive immune response can be evoked in an automated manner from a single cell by TLR signals, and that the only mode of regulation of this system is whether cells are stimulated above a threshold to progress through successive divisions. In marked contrast to the two innate stimuli, many of the quantitative attributes of the B-cell response to CD40 stimulation can be tuned in a graded manner. This is particularly striking for division times: where changing the concentration of LPS and CpG altered the proportion of cells undergoing first division, and changing the concentration of CD40 stimulation modified the time to the first division. The other marked difference was in the rate of differentiation to ASC. Although this was an autonomous, constant function of the LPS response, the rate of generation of ASC was regulated by CD40 stimulation strength, with low concentrations giving a higher proportion of differentiation per cell. This finding, in conjunction with recent studies illustrating that asymmetric inheritance of antigen by B cells in vivo directly regulates interaction levels with helper T cells [20] , identifies that the level of CD40 stimulation has an integral, but complex, role in allocation of B cells to distinct effector lineages during humoral immune responses. Although CD40-stimulated B cells appear receptive to complex modulation by external signals, they do still possess some features of autonomous control. If the stimulus is removed before first division, some of the stimulated cells will continue to divide [22] , [36] and undergo division-linked isotype switching [16] , [36] . For these reasons, we envisage this more evolutionarily recent form of antibody regulation as a hybrid, building on a framework of automated behaviour while taking inputs from many sources to alter the outcome. We also point out that for all stimuli used, their removal from culture resulted in less overall cell division, suggesting that degradation or loss of potency of the stimuli under these culture conditions was not a significant influence on the outcome [22] , [36] . We consider it noteworthy that the autonomous TLR-mediated mode of regulation is driven by a family of evolutionarily ancient proteins [37] . Homologues for key components of the Toll signalling pathway are found to have an important role in immune function in species as diverse as plants, Drosophila , mouse and human [38] . In contrast, the acquisition of genetic components that facilitated the development of the adaptive immune response, which relies heavily on TD signals, has occurred more recently [39] . Thus, we speculate that the earliest form of immune responses, and perhaps those still used by simple organisms, operates using the directly proportional activation and fate allocation mechanism. In contrast, in the more advanced TD system, the default antibody response is weaker but capable of integrating multiple additional inputs that alter the quantitative outcomes. Finally, our study highlights a key advantage of using a probabilistic approach to account for the intrinsic heterogeneity in B-cell populations in response to stimulation—identification of the molecular basis for the variation is not necessary for our model to accurately portray the outcome. Nevertheless, we suggest this variation arises from the typical lognormal variation in cellular expression of receptors and signalling intermediates, which itself derives from stochasticity and epigenetic modification of gene expression [40] , [41] , [42] , [43] . 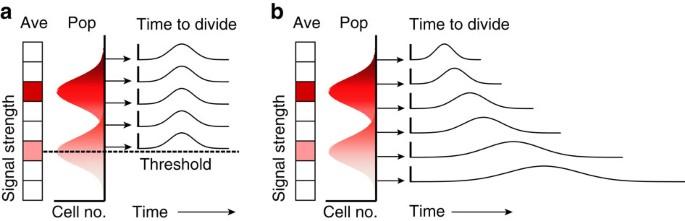Figure 7: Two patterns for heterogeneity in the population. In (a), the quantal response of CpG and LPS stimulation is illustrated. For a high- and low-stimulation level (Ave), the actual graded variation in signalling in the population is shown (Pop). This gradation leads to half the cells falling below the threshold for proliferation in the lower stimulation dose. However, for all cells above the threshold, the times to divide show a similar range of variation, unaffected by stimulation dose, or ranking in population sensitivity. (b) The graded response to CD40 stimulation. Here the times to divide are proportional to the stimulation level, whether altered by concentration of ligand or inherent sensitivity in the population. Figure 7 summarizes our interpretation of the heterogeneity differences in signal processing by TI versus TD receptors. For TLR signals, once a threshold is reached, the sensitivity of the population and level of signal regulates recruitment to an automated antibody response ( Fig. 7a ). In contrast, altering the concentration of CD40 stimulation, or sensitivity of the population to this input, influences both division times and differentiation ( Fig. 7b ). However, in both cases, the response of cells with low intrinsic sensitivity is equivalent to cells with high sensitivity exposed to lower ligand concentrations ( Fig. 7 ). We argue that although this response is highly predictable at the population level, the net result of this variation is unique for each responding B cell and its progeny, and this heterogeneity is pivotal in the allocation to multiple effector lineages [23] . Figure 7: Two patterns for heterogeneity in the population. In ( a ), the quantal response of CpG and LPS stimulation is illustrated. For a high- and low-stimulation level (Ave), the actual graded variation in signalling in the population is shown (Pop). This gradation leads to half the cells falling below the threshold for proliferation in the lower stimulation dose. However, for all cells above the threshold, the times to divide show a similar range of variation, unaffected by stimulation dose, or ranking in population sensitivity. ( b ) The graded response to CD40 stimulation. Here the times to divide are proportional to the stimulation level, whether altered by concentration of ligand or inherent sensitivity in the population. Full size image Cohort analysis The cohort analysis method has been described previously [27] . Briefly, precursor ‘cohort’ data are produced by removing the effect of cell expansion. We begin with a set of cell population data giving the number of cells in each division at a series of time points. This cell population data are transformed into cohort data simply by dividing the cell population number by two to the power of the division number (undivided cells are considered to be in division 0), and this removes the effect of clonal expansion on the data. For each time point, we fit the cohort profile for all divisions ( n >0) to a function of the form Where is a normal distribution with mean μ and s.d. σ . The parameter γ ( t ) is the cohort size, whereas μ div ( t ) and σ div ( t ) are the mean and s.d. division number of the cohort as a function of time. From these parameters, we can extract the mean time to first division μ 0 and the time to subsequent divisions τ from the following relation: thus, by plotting the mean division number, as determined using the above technique, at various time points against time, we obtain a linear plot with a gradient equal to 1/ τ . In practice, this plot will only be linear during the expansion phase of the B-cell response, when the cells are proliferating without significant death. As the cells cease proliferating and start to die, the plot will flatten out. Therefore, we must identify a set of time points for which the cells have proliferated enough to provide a reliable fit to their cohort division profile; typically this requires a mean division number , and before a significant fraction of the cells have ceased proliferation. To these points, we fit a straight line, and from this line we determine the subsequent division time, from the inverse gradient, and the mean time to first division. The mean time to first division is the time at which , which is determined by extrapolation from the linear fit. The cohort method can also give an indication of the amount of death that occurs as cells progress through subsequent divisions. The parameter γ ( t ), the cohort number, used to weigh the distribution in the fit to the cohort plots, represents the total number of the original cohort of dividing cells surviving at each time point. This parameter is sometimes referred to as the cohort area, as it represents the total area of the weighted normal distribution that is used in the fit to the cohort plot. Therefore, if the cohort number remains constant through a set of time-course data, there is little or no death. If the number is decreasing as the time-course progresses, some cells are being lost to death. The pattern of loss in this line will give an indication of the amount of death per division during a time course. Confidence limits in the cohort analysis Confidence limits in the cohort analysis were obtained using a bootstrap procedure [44] whereby the data set of n replicates was re-sampled with replacement to obtain a new pseudo-data set of the same dimension. Each time point was re-sampled independently as different time points are statistically independent. This re-sampling was performed a total of N =100 times, and an identical cohort analysis performed on the re-sampled data, yielding a set of N parameter estimates. The lower and upper limits of the 95% confidence intervals quoted are the values for which 97.5% of the re-sampled estimates lie above and below, respectively. Cyton analysis The cyton analysis presented in this work has been performed by fitting the cyton model, as outlined previously [21] , to division structured population data. Briefly, for each stimulus analysed, we fit the model to all concentrations simultaneously, allowing different sets of parameters to vary concentration stimulus. Each concentration represents a separate time course, and hence requires a separate parameterization of the model. There are 12 parameters associated with the model if the starting cell number is considered as a separate parameter, and thus if we have N stimulus concentrations, we have a maximum of 12 N free parameter values to obtain. In this work, we have always set the starting cell number to be constant across all concentrations, which gives a maximum of 12+11( N− 1) parameters. However, for many fits, we place constraints on other parameters, requiring that they too are equal for all divisions, thus further reducing the number of free parameters. We fit to the experimental division structured population data using a weighted sum of least squares approach where we minimize: Here n i,j,k,l is the measured number of cells in the i th division at the j th time point, the k th replicate and the l th concentration. The value y i,j,k represents the model prediction for the number of cells at the same point, and there is no need to include a index for replicate here as the model prediction is the same for all replicates. We include a contribution ε =13.8 (the average value obtained from linear fits of the variance to the mean for the three data sets) in the denominator to remove underflow errors when the model predicts zero cells at a point, which can be thought of as a lower bound of the variance of the experimental noise. We have used this least squares metric for fitting models to the data and have used the AIC to compare the quality of fits between different models. An alternative approach would be to fit using quantities such as the Kulber–Leibler divergence [45] or the Bhattacharya distance [46] that represent information measures and would allow direct comparison between models. The fitting is performed using the MATLAB routine fmincon (Mathworks, Natick, MA) to minimize the value of χ 2 for a given set of experiments. Briefly, we fit our model by minimizing the sum of square residuals between predicted and measured cell numbers, weighted by the predicted cell number. Here the weighting counters the tendency of the metric to give less weight to points with fewer cells and is consistent with the observation that the variance in measurement between replicates generally increases with the average measurement. As such, we have adopted the approach outlined in Leon et al. [47] where a small offset is added to this weighting to prevent divergence of the measure at points for which the model predicts a vanishing number of cells. Because of the broadening of the CFSE peaks with increasing division, we have assigned an upper division of 7 to both our model and experimental data, such that division number 7 (undivided cells are given a division number of 0) will include all cells in division 7 and higher. Akaike information criterion We compare models with different numbers of parameters using the AIC, calculated in the following way [48] : here RSS is the residual sum of squares of the model fit to the data, k is the number free parameters in the model and n is the number of observables that have been fit to. In general, a better fit to experimental data (reduced value of RSS ) can be achieved by increasing the number of parameter of the model. The AIC protects against over-fitting by applying a penalty for adding more parameters to the model. Mice Female C57BL/6 mice 6–18 weeks of age were used for all experiments. Blimp-1 mice were provided by Professor Steve Nutt (Walter and Eliza Hall Institute (WEHI)). All animals were bred at the WEHI animal facility (Kew, Victoria, Australia) and were maintained in specific pathogen-free conditions at WEHI (Parkville) in accordance with WEHI animal ethics committee regulations. B-cell isolation and cell culture Single-cell suspensions were prepared from spleens of mice, red cells lysed and run on discontinuous percoll density gradients. Small dense cells were collected from the 65–80% interface and B cells purified via negative selection using magnetic bead B-cell isolation kits (Miltenyi Biotec, Auburn, CA). For division-tracking experiments, cells were labelled with CFSE according to the method described below. B cells were typically >95% B220+, CD19+, IgM+ and IgD+ as determined by flow cytometry. B cells were cultured and stimulated in B-cell medium comprising RPMI 1640 medium (Gibco BRL) with 2 mM L -glutamine, 1 mM Na-pyruvate, 0.1 mM nonessential amino acids, 10 mM HEPES, pH 7.4, 100 μg ml −1 of streptomycin, 100 U ml −1 of penicillin, 50 μM β-mercaptoethanol (all supplements were purchased from Sigma) and 10% heat-inactivated FCS (CSL, Parkville, Victoria, Australia). B cells were stimulated with the indicated concentrations of the following reagents. LPS from Salmonella typhosa (Sigma). Recombinant mouse IL-4 was a gift of R. Kastelein (DNAX Research Institute, Palo Alto, CA) and supplemented at a saturating concentration of 1000 U ml −1 . The α-CD40 antibody (1c10) was prepared from the original hybridoma [33] provided by DNAX Research Institute. CpG DNA oligonucleotide CpG-1668, fully phosphorothioated (sequence, 5′-TCCATGACGTTCCTGATGCT-3′; Geneworks, Adelaide, South Australia, Australia). CFSE labelling Intracellular proteins within lymphocytes were CFSE-labelled for division-tracking experiments according to the protocol described previously [49] . Briefly, B cells were washed once in PBS/0.1% BSA and resuspended at 1 × 10 7 ml −1 . A 5 mM stock of carboxyfluorescein diacetate succinimidyl ester (Molecular Probes, Eugene, OR) was diluted 1/10 with PBS/0.1% BSA. Diluted stock of 20 μl was added per ml of cells for a final concentration of 10 μM. Cells were incubated at 37 °C for 5 min, mixed thoroughly by vortexing and incubated for another 5 min. CFSE protein labelling was stopped by adding 10 volumes of ice cold RPMI/10% FCS. Flow cytometry To determine absolute cell numbers, the number of live cells per culture was estimated by reference to a known number of Calibrite beads (Becton Dickinson, San Jose, CA), added directly to cell culture before collecting. Cell numbers were calculated using the following formula: Dead cells were identified via addition and uptake of propidium iodide (Sigma Aldrich) also added before collecting. For differentiation analysis, collected cells were spun down and washed once in PBS+2% FCS. Cells were stained for 30 min at 4 °C with anti-syndecan-1 (CD138) antibody (BD Pharmingen, San Jose, CA) conjugated to phycoerythrin at a dilution of 1/500. Flow-cytometric data were collected on FACScan or LSR flow cytometers (BD Biosciences) and analysed with Flow-Jo software (Tree Star). Colcemid analysis For direct analysis of time of entry into first division, cells were stimulated in the presence of 25 ng ml −1 colcemid (Roche, Indianapolis, IN). Cultures were pulsed with 1 μCi per well [methyl- 3 H] thymidine (Amersham Biosciences, UK) for 1 h before collecting. Incorporation of radioactivity was measured using a scintillation counter (Topcount NXT; Packard, Meridan, CT). How to cite this article: Hawkins, E. D. et al. Quantal and graded stimulation of B lymphocytes as alternative strategies for regulating adaptive immune responses. Nat. Commun. 4:2406 doi: 10.1038/ncomms3406 (2013).